Myogenin promotes myocyte fusion to balance fibre number and size Each skeletal muscle acquires its unique size before birth, when terminally differentiating myocytes fuse to form a defined number of multinucleated myofibres. Although mice in which the transcription factor Myogenin is mutated lack most myogenesis and die perinatally, a specific cell biological role for Myogenin has remained elusive. Here we report that loss of function of zebrafish myog prevents formation of almost all multinucleated muscle fibres. A second, Myogenin-independent, fusion pathway in the deep myotome requires Hedgehog signalling. Lack of Myogenin does not prevent terminal differentiation; the smaller myotome has a normal number of myocytes forming more mononuclear, thin, albeit functional, fast muscle fibres. Mechanistically, Myogenin binds to the myomaker promoter and is required for expression of myomaker and other genes essential for myocyte fusion. Adult myog mutants display reduced muscle mass, decreased fibre size and nucleation. Adult-derived myog mutant myocytes show persistent defective fusion ex vivo. Myogenin is therefore essential for muscle homeostasis, regulating myocyte fusion to determine both muscle fibre number and size. Regulation of tissue size requires balancing cell number and cell size. In skeletal muscle, tissue size depends on generating the correct number of multinucleated muscle fibres with an appropriate number of nuclei in each; how these processes are controlled in vertebrates is mysterious. Formation of syncytial muscle fibres is a three-step process: commitment as a myoblast, terminal differentiation into a myocyte, defined here as irreversible cell cycle exit and expression of muscle-specific actin, myosin and other genes, and finally myocyte fusion and growth to form a mature multinucleate myofibre. In specialised circumstances, such as the mononucleate slow myofibres of larval zebrafish, myocytes mature into functional innervated and contractile muscle fibres without fusion. The Myogenic Regulatory Factor (MRF) family of transcription factors (Myod, Myf5, Mrf4 and Myog) are key players in orchestrating each of these steps in skeletal myogenesis [1] , [2] . All MRF genes encode a basic domain and Helix–Loop–Helix (bHLH) motif, which account for protein–DNA binding and hetero-dimerization with ubiquitous E-proteins, respectively, by which they activate expression of many E-box-containing muscle-specific genes [3] , [4] . Whereas three MRFs drive myoblast formation during early development, Myog acts later to regulate myoblast terminal differentiation, myofibre maturation and size [1] , [2] . Genetic studies in mice revealed that among MRFs only Myog is essential for viability; null Myog mutation leads to perinatal death, due to severely defective muscle differentiation, although residual differentiated muscle fibres are present [5] , [6] , [7] , [8] . Absence of Myog does not prevent slow and fast fibre type diversification [7] , [8] . In vitro studies on primary myoblasts or embryonic stem cells from Myog mutant mice reveal terminal differentiation comparable to wild-type (wt) albeit yielding smaller syncytial myotubes [6] , [7] , [8] , [9] , [10] , suggesting that extracellular factors determine the need for Myog function. Congruently, Myog −/− myoblasts efficiently contribute to multinucleated fibres in genetic mosaic experiments [11] . Furthermore, depletion of Myog after birth reduces myofibre size and affects overall body homeostasis, although without perturbing muscle histology [12] , [13] , [14] . However, given that other MRFs can and do bind the same DNA motifs as Myog [15] , the precise role(s) of Myog remain ill-defined. Knockdown of zebrafish myog has minor effects on initial events in myogenesis [16] , [17] , [18] , [19] , whereas combined knockdown of Myog and Myod strongly reduces myogenesis of fast myofibres [17] . These findings were confirmed using a zebrafish mutant ( myog fh265 ) bearing a stop mutation downstream of the bHLH domain, which also shows delayed muscle regeneration [18] , [20] . However, as a similar truncation of mouse Myog has residual activity, we previously suggested that myog fh265 is hypomorphic [18] , [21] . Hence, despite strong evidence for roles for Myog in later myogenesis not compensated for by other MRFs [7] , [8] , a specific evolutionarily-conserved function in vivo is unclear. Here we create null alleles in zebrafish myog and reveal a specific function for Myog in myocyte fusion during skeletal muscle development. We find that Myog is dispensable for myoblast terminal differentiation, expression of many muscle-specific markers, myofibre elongation across the somite, sarcomere assembly, innervation and generation of functional contractile muscle. However, lack of Myog prevents most myocyte fusion and leads to supernumerary mononucleated muscle fibres. Myog is required for the expression of membrane proteins involved in cell fusion, such as Myomaker [22] , [23] , [24] , [25] . Despite gross myocyte fusion defects, zebrafish myog mutants survive to adulthood with more but thinner muscle fibres and reduced overall body size. Adult muscle precursor cells lacking Myog show a persistent fusion defect ex vivo. Interestingly, residual fusion in myog mutants occurs primarily in the deep myotome and is dependent upon Hedgehog signalling, indicating the existence of two pathways to myocyte fusion. Generation of myogenin mutant alleles To create a null myog mutant, we targeted genome editing far upstream of bHLH region and obtained two nonsense alleles (Fig. 1a ). Myog kg128 has an insertion of 1 bp (A), whereas myog kg125 has a deletion of 3 bp (TCA). Both mutations create a stop codon in an identical position (Y37*), producing a truncated protein lacking both basic and HLH domains. In situ mRNA hybridisation (ISH) for myog on myog kg128/+ and myog kg125/+ incross lays at 18 h post fertilization (hpf) showed reduced signal in mutant embryos compared to siblings (sibs), presumably by nonsense-mediated decay (NMD) (Fig. 1b ). mRNA downregulation was confirmed by qPCR at 20 hpf (Fig. 1c ). Congruently, mutant embryos lacked Myog immunoreactivity, whereas F-actin accumulation and overall number of nuclei per myotome was indistinguishable from wild-type (wt) (Fig. 1d ). Heterozygote and wt siblings showed similar levels of Myog (Supplementary Fig. 1a ). No compensatory upregulation of other MRFs was noted at 20 hpf. Indeed, lack of Myog significantly reduced expression levels of myf5 (40%) and mrf4 (54%), whereas myod remained unchanged (Fig. 2a ). These results demonstrate that homozygous mutant alleles myog kg125 or myog kg128 block Myog mRNA and protein accumulation. Fig. 1 Genome editing generates zebrafish myog null alleles. a Schematic of myog gene exons (boxes) and protein showing the position of kg125 , kg128 and fh265 mutant alleles. The tyrosine to stop mutations (Y37*) produce a truncated protein of 36 amino acids (aa) devoid of both basic (yellow) and helix–loop–helix (HLH, green) domains. The fh265 hypomorphic allele (Q167*) truncates downstream of bHLH. Beneath, DNA and protein alignment of wild-type (wt), 3 bp kg125 deletion (red) and 1 bp kg128 insertion (green) alleles with novel stop codons underlined causing an identical truncation. b In situ mRNA hybridisation (ISH) for myogenin on myog kg128/+ and myog kg125/+ incross lays reveal NMD of mutant myog mRNA at 20 somite stage (20 ss). Representative images n = 14 + 5 mutants, n = 39 + 22 sibs, respectively. Insets show magnification of boxed areas. c qPCR analysis on wt sibs and myog kg125 embryos at 22 ss confirms NMD. Mean fold change ± SEM from four independent experiments on genotyped embryos from four separate lays analysed on separate days, paired t test statistic. Symbol shapes denote matched wt and mutant samples from each experiment. d Immunoreactivity of Myog is lost in myog kg125 and myog kg128 mutants at 20 ss, whereas F-actin is unaffected. Insets show nuclear staining in myog kg125 and sib using Hoechst counterstain. Relative myotomal Myog immunofluorescence was assessed by nuclear intensity measurement. All images are lateral views anterior to left, dorsal to top. Representative images n = 10 + 7 mutants, n = 9 + 19 sibs, respectively. Bars = 50 µm Full size image Fig. 2 Functional muscle differentiation in Myogenin mutants. a qPCR analysis on wt sibs and myog kg125 embryos at 22 ss showing reduction of myf5 , mrf4 but not myod RNAs. Mean fold change ± SEM from four independent experiments on genotyped embryos from four separate lays analysed on separate days, paired t test statistic. Symbol shapes denote matched wt and myog mutant samples from each experiment. b , c Immunodetection of slow and fast myosins (sMyHC and fMyHC) in 2 dpf larvae from a myog kg125/+ incross showing that myofibre differentiation occurs in mutant. Dots in graphs show slow myofibre width (average of six myofibres/larva) and number in somite 17 of sib and mutant individuals. Representative images n = 5 mutants, n = 8 sibs. d – f Phalloidin staining for F-actin or immunolabelling for titin and α-actinin reveals that mutant myofibres display regular sarcomere spacing and are properly assembled to sustain contraction. Representative images n = 5 mutants, n = 21 sibs (phalloidin); n = 7 mutants, n = 18 sibs (titin); n = 7 mutants, n = 23 sibs (α-actinin). In f , boxes are shown magnified below. g Sarcomere length from f (average of 6 myofibres/larva) in sibs and mutants. Numbers of larvae analysed are shown on columns ( b , g ). h Larvae from a myog kg128/+ incross stained with α-bungarotoxin-Alexa-488 show that mutant embryos accumulate AChR at both neuromuscular junction (arrows) and muscle-muscle junction (arrowheads) comparable to sibs. Representative images n = 4 mutants, n = 11 sibs. i Motor function of 5 dpf larval zebrafish in fish-water (FW; n = 24 mutants, n = 115 sibs) or 0.6% Methyl-Cellulose (MC; n = 12 mutants, n = 36 sibs) as time spent moving (minutes), distance travelled (mm) and average speed (mm/s). Overall muscle function is unaffected by lack of Myog in both FW and MC. Activity of both myog mutants and sibs is affected by MC. Each dot represents the behaviour of an individual larva. ns: not statistically significant in ANOVA. Bars = 50 µm (10 µm in g ) Full size image Myoblasts differentiate and muscle functions without Myogenin To examine muscle differentiation, mutants and sibs were compared for mylpfa and smyhc1 expression that distinguish fast and slow muscle [26] , [27] , [28] . ISH analysis revealed no difference at 15 somite stage (ss) (Supplementary Fig. 1b ). In this and subsequent experiments, no differences were observed between wild type and heterozygous sibs, consistent with their similar Myog level (Supplementary Fig. 1a ). At 22 ss, strong mylpfa mRNA in fast muscle in anterior somites and smyhc1 mRNA in slow muscle extending more posteriorly were also unaltered in myog mutants (Supplementary Fig. 1c ). At this stage, slow myofibres have migrated to the lateral surface of the myotome and remain mononucleated, whereas the more abundant multinucleated fast muscle fibres are located deeper in the myotome [29] , [30] , [31] . Moreover, no obvious difference was observed, either in motility or in fast and slow myosin heavy chain (MyHC) immunoreactivity at 20 hpf, 1 day post-fertilisation (dpf) or 2 dpf, when embryos have hatched and make short bursts of controlled swimming (Fig. 2b,c and Supplementary Fig. 1c-e ). Slow myofibre number and thickness were not affected in mutants (Fig. 2b and Supplementary Fig. 1e ). Thus, without Myogenin, specification and early development of slow and fast muscles appears normal. α-Actinin, Titin, F-actin and Acetylcholine Receptor staining also showed that fibre formation, sarcomere assembly and innervation had occurred properly in mutants (Fig. 2d–h ). At 2 dpf, mutant myofibres were correctly positioned and elongated across the length of the somite. However, fast muscle appeared mildly disorganised and slightly reduced in extent (Fig. 2f ). Nevertheless, motor function at 5 dpf assayed by time spent swimming, total travelled distance and average speed did not differ between myog mutants and sibs. Irrespective of genotype, some larvae were consistently more active than others throughout the 30 min measurement period (Fig. 2i ). To test fibre integrity and anchorage, fish were swum in a viscous methyl-cellulose (MC) solution, which led to a general decrease of swimming performance. Despite this challenging environment, mutants did not perform significantly worse than their siblings (Fig. 2i ). When sib and mutant larvae were grown in MC from 5 to 8 dpf, a procedure known to damage defective muscle [32] , myog mutants retained good muscle morphology (Supplementary Fig. 1f ). Thus, Myogenin is dispensable for the initial phases of myogenesis and generation of strong functional muscle in zebrafish. Muscle size reduction and myofibre number increase in myog mutant Although functional muscle was formed, our data suggested a reduction in myotome size in mutants (Fig. 2 ). Measurement of the dorso-ventral extent of ISH staining of fast mylpfa and slow smyhc1 revealed a reduction of mutant myotome size, both at 1 and 2 dpf (Fig. 3a, b and Supplementary Fig. 2a ). Nevertheless, the body length of mutants and sibs was comparable, suggesting that muscle reduction was not due to reduced overall body size or delayed development (Fig. 3c and Supplementary Fig. 2b ). Fig. 3 Myogenin is required for normal larval muscle growth. a , b ISH for mylpfa mRNA showing similar level of expression of fast myosin but reduced extent of somitic muscle in mutants ( a , red brackets) at 1 and 2 dpf. Myotome height ( b ) is significantly reduced in myog kg128 mutants at 1 and 2 dpf. Representative images n = 9 + 18 mutants, n = 35 + 63 sibs. c Larval length is unaffected in mutant at 2 dpf, showing that muscle reduction is not due to overall reduced size of mutant larvae. d Schematic of myotome volume measurement. β-actin : EGFP ; myog kg128/+ fish were incrossed and progeny imaged by confocal microscopy. Lateral and three equi-spaced transverse images of somite 17 were collected from each larva at each stage (dashed lines). Transverse area (red outline) multiplied by somite length (cyan dashed line) yielded myotome volume for each fish at each stage. e Optical transverse-sections of β-actin : EGFP ; myog kg128 mutants show reduced myotome area at 2, 3 and 5 dpf compared to sibs (dashed red lines). Boxes are shown magnified beneath highlighting smaller fibre cross-sections in mutants (dashed white lines). Representative images n = 6 mutants, n = 14 sibs (2 dpf); n = 5 mutants, n = 18 sibs (3 dpf); n = 9 mutants, n = 13 sibs (5 dpf). f Myotome volume reduction in myog kg128 mutants at 2, 3 and 5 dpf. g – i . Myotome length ( g ), number of fast fibres per cross section ( h ) and fibre volume ( i ) at 2 dpf compared by t tests. Bars = 50 μm. nt: neural tube, nc: notochord Full size image To analyse the defect in cellular detail, myog kg128 and myog kg125 were bred onto Tg(Ola.Actb:Hsa.HRAS-EGFP) vu119 , in which EGFP targets plasma membranes of all cells [33] ( β-actin:EGFP hereafter). Confocal sections of β-actin : EGFP ; myog kg128/+ incross larvae confirmed that reduction in myotome volume was present at 2 dpf in mutants and persisted until at least 5 dpf (Fig. 3d, f ). Although myotome cross-sectional area was consistently reduced in mutants, myotome length was unaffected (Fig. 3g ; Supplementary Fig. 2b ). A reduction of fast fibre cross-sectional area in mutant fish was observed (Fig. 3e ). Indeed, quantitative analysis at 2 dpf revealed a 50% increase of fast fibre number accompanied by a 45% reduction in mean fibre volume in mutant embryos (Fig. 3h, i ). myog fh265 mutants did not have reduced size or altered cellularity and we did not observe any other phenotype in un-manipulated embryos, larvae or adults, confirming that this allele is hypomorphic [18] (Supplementary Figs 2 c–e; 5a ). We conclude that Myog controls fast myofibre number and size. Myogenin is required for normal myocyte fusion Two hypotheses could explain the overabundance of fast muscle fibres in myog kg128 and myog kg125 mutant embryos: increased frequency of terminal differentiation of muscle progenitor cells (MPCs) into myocytes or reduced fusion of differentiating myocytes into multinucleate fibres. Most, if not all, fast myofibre nuclei derive from MPCs expressing either Pax3 or Pax7 [34] , [35] , [36] , [37] , [38] , [39] , [40] , [41] , [42] . We found no differences between myog mutants and sibs in position or number of Pax3/7 positive cells at 1–2 dpf (Fig. 4a, b ). Nor was there a change in the number of nuclei in the myotome (Fig. 4h ). Thus, no evidence supported the possibility that myocyte formation from MPCs was increased. Fig. 4 Myogenin promotes fusion of myocytes. a , b Immunodetection and quantification of Pax3/7 positive MPCs in somite 17 of myog kg125/+ incross embryos at 1 dpf and 2 dpf. Mean ± SEM of dots representing individual embryos. Lack of Myog does not alter number of Pax3/7 MPCs per somite (white dashed lines). Representative images n = 6 mutants, n = 11 sibs (1 dpf); n = 8 mutants, n = 9 sibs (2 dpf). c Qualitative analysis of myoblast fusion in a myog kg125/+ incross injected at 1-cell stage with DNA encoding CAAX-membrane targeted mCherry (red). At 2 dpf, larvae were fixed and stained with Hoechst to highlight nuclei (blue) and analysed from 3D stacks. Nuclei within mCherry-labelled fibres (arrowheads) were mostly single in mutants, but multiple in sibs. Representative images n = 6 embryos. d Myoblast fusion quantified by injection of H2B:mCherry RNA into 1-cell stage embryos from β-actin:EGFP;myog kg128/+ incross. Confocal single plane images deep in the myotome of 2 dpf larvae showing muscle fibres and the position of nuclei (insets). Note the central location away from somite borders (dashed white lines) of most nuclei in mutants (arrowheads), similar to that observed in mononucleate superficial slow fibres. Representative images n = 6 embryos. e , f Quantification of fusion within the entire myotome 17, showing the fraction of fast fibres ( e ) and fraction of nuclei in fast fibres ( f ) with the indicated number of nuclei. Slow fibre numbers were unaltered. Data report mean values of three larvae per genotype (see Supplementary Fig. 3a for individual data). p -values indicate probability of rejecting null hypothesis of no difference between mutant and sibs in χ 2 tests. g Number of nuclei per fast fibre is reduced in mutant. h Total number of nuclei within fast fibres in somite 17 of sib and mutant is unchanged. Dots represent individual embryos. Mean ± SEM. t test. Bars = 50 μm. i , j Mosaic myog:MyogCDS-IRES-GFP plasmid-derived expression of Myog (Myog O/E) rescues fusion in myog kg128 mutant larvae from a myog kg128/+ incross, compared control myog:GFP plasmid (Control). Quantification (as in e ) of nuclei in GFP + cells ( i , see Supplementary Fig. 4a for individual data). Immunodetection shows Myog overexpression (Myog O/E, magenta) in myog:MyogCDS-IRES-GFP but not in myog:GFP (Control, green) GFP + fibres ( j ). Representative images n = 5 myog:GFP , n = 11 myog:MyogCDS-IRES-GFP injected mutants, ns: not significant Full size image Next, we tested the ability of Myog to promote myocyte fusion. We injected DNA encoding CAAX-mCherry at the 1-cell stage into myog kg128/+ incross embryos to label mosaically the plasma membrane of single fibres. At 2 dpf the majority of labelled fibres in mutant embryos were mononucleated, whereas those in sibs were multinucleate (Fig. 4c ). To quantify this defect, we injected H2B-mCherry mRNA into β-actin : EGFP ; myog kg125 embryos to label nuclei and plasma membranes uniformly. Strikingly, over 92% of muscle fibres in myog mutants were mononucleate, compared to 33% in sibs (Fig. 4d, e ; Supplementary Fig. 3a ). The fraction of nuclei in multinucleate fibres dropped from 81% in sibs to 16% in mutants (Fig. 4f ; Supplementary Fig. 3a ). This phenotype persisted at least until 6 dpf (Supplementary Fig. 3b ). Nuclei in mononucleated myofibres preferentially located near the centre of the myotome (Fig. 4d ). Despite the twofold reduction in myonuclei per myofibre, the total number of nuclei within in each myotome was not altered in mutants, paralleling the increase in myofibre number (Figs. 3 h; 4g, h ). To eliminate the possibility of CRISPR off-target effects, we re-expressed Myog mosaically in myog mutant larvae by injection of a plasmid containing the zebrafish myog promoter driving wt zebrafish Myog-IRES-GFP expression. myog:MyogCDS-IRES-GFP rescued fusion in fast fibres, whereas a control myo g:GFP -only vector did not (Fig. 4i, j ). Myog knockdown with a morpholino fully recapitulated the mutant phenotype with increased number of mononucleate fibres and decreased somite growth (Supplementary Fig. 3c–e). We conclude that Myogenin is essential for most myocyte fusion. To examine the cell autonomy of the need for Myogenin we analysed myog mutant larvae with mosaic Myog-IRES-GFP re-expression further. Myog-IRES-GFP significantly rescued fusion; Myog-expressing fibres in myog mutants contained a range of nuclear numbers approaching the distribution in controls (compare Fig. 4e, i ). Adjacent unlabelled fibres remained mononucleate (Fig. 4j ). As cells expressing Myog-IRES-GFP occurred at a rate of about 2–3 per somite and were well-scattered, this finding indicates that only a single fusing partner needs to express Myog to permit fusion. Moreover, although mosaic Myog expression rescued mutants, it did not induce more fusion than observed in wt in either mutants or sibs (Fig. 4i, j ; Supplementary Fig. 4a–c ). Importantly, Myog expression (either in myog mutants or sibs) failed to elicit fusion of the normally-mononucleate slow fibres, even though the slow fibres were adjacent to fast fibres and their MPC precursors, indicating that the low level of myog mRNA in wt slow MPCs is not the only reason for their lack of fusion (Supplementary Fig. 4d,e ). However, both mutant and sib slow fibres overexpressing Myog-IRES-GFP showed significantly reduced myofibrillar width (Supplementary Fig. 4e,f ). Thus, Myog is required in at least one of two fusing fast myocytes to permit fusion. Expression of fusogenic genes reduced in myog mutants Fusion of myocytes is a key feature of skeletal myogenesis and requires several transmembrane proteins [43] . We hypothesised that Myog regulates these genes. Myomaker ( mymk ) [22] , [23] , [24] , [25] , [44] mRNA was strongly reduced (72%) in myog null mutant embryos at 20 hpf, during initial myocyte fusion, and was also mildly affected in myog fh265 hypomorphs (Fig. 5a, b ; Supplementary Fig. 5a ), paralleling the previously observed myog nonsense-mediated mRNA decay in this hypomorphic allele [18] . Mymk was also reduced in myod fh261 mutant in proportion to myog mRNA reduction and loss of fast muscle [18] , [45] (Supplementary Fig. 5a,b ). Reduction of mymk mRNA thus parallels lack of myocyte fusion. Myomixer/myomerger/minion , a micropeptide recently described to enhance myoblast fusion [44] , [46] , [47] , was also reduced (34%; Fig. 5b ). Moreover, jam3b mRNA was significantly reduced (22%) in mutants, but jam2a [48] and kirrel3l [49] were unaffected (Fig. 5a, b ). Fig. 5 Myogenin mutants have reduced expression of fusogenic factors. a ISH on 20 hpf myog kg128/+ incross to investigate the expression of genes essential for vertebrate myocyte fusion. Expression of myomaker ( mymk ) and jam3b , but not of jam2a or kirrel3l , is reduced in myog mutant. Bar = 50 μm. Representative images n = 10 mutants, n = 38 sibs ( mymk ); n = 13 mutants, n = 37 sibs ( jam2a ); n = 12 mutants, n = 39 sibs ( jam3b ); n = 7 mutants, n = 13 sibs ( kirrel3l ). b qPCR analysis of RNA expression levels showing downregulation of mymk , myomixer/myomerger/minion ( mymx ) and jam3b at 20 hpf on myog kg125 mutants, whereas jam2a and kirrel3l remain unaltered compared to wt ( myog +/+ ) sibs. Graphs show mean fold change ± SEM of four independent experiments; paired t test. Symbol shapes denote wt and mutant samples from paired experiments. c Schematic of 5' genomic region of mymk reporting: 5′-UTR and coding sequence (grey and white boxes), position of E-box elements (red boxes), relative bp distance from 5'UTR start (+1), start codon (arrow, ATG). E-box 1 and E-box 2 sequences are shown in red text. d ChIP-qPCR assay using anti-Myog or mock showing significant Myogenin enrichment on mymk E-box 1 compared to negative controls from the gapdh promoter and a gene-free region on chromosome 14 containing an E-box (Chr14). Mean of percentage of input immunoprecipitated ± SD of two independent experiments, ANOVA Full size image The extent of reduction of myomaker expression in mutants argues for direct transcriptional regulation by Myogenin. To test whether Myog directly regulates mymk transcription in zebrafish, we scanned 3 kb of putative promoter region upstream of the myomaker 5'-UTR and found two E-box elements (E-box 1 and E-box 2, Fig. 5c ). ChIP-qPCR assay on 20 hpf embryos revealed that endogenous Myog binds both E-box elements, with significant enrichment of Myog enin binding to E-box 1 compared to two different negative controls. The more proximal E-box 1 showed greater binding than E-box 2 (Fig. 5d ). Combined, these data support a role for Myogenin in governing myocyte fusion through direct transcriptional upregulation of mymk and other fusogenic factors. Hedgehog drives residual fusion and mymk expression Myog mutants retain small numbers of multinucleate fibres in the medial somite (Fig. 4e ; Supplementary Fig 3a,b ). Residual mymk mRNA also persists in myog mutants (Fig. 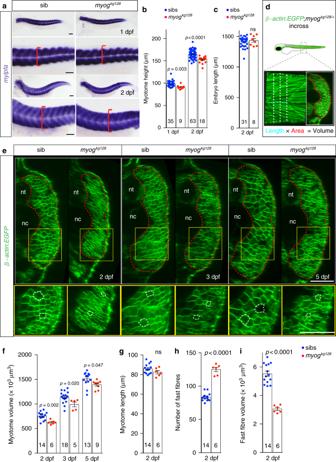Fig. 3 Myogenin is required for normal larval muscle growth.a,bISH formylpfamRNA showing similar level of expression of fast myosin but reduced extent of somitic muscle in mutants (a, red brackets) at 1 and 2 dpf. Myotome height (b) is significantly reduced inmyogkg128mutants at 1 and 2 dpf. Representative imagesn= 9 + 18 mutants,n= 35 + 63 sibs.cLarval length is unaffected in mutant at 2 dpf, showing that muscle reduction is not due to overall reduced size of mutant larvae.dSchematic of myotome volume measurement.β-actin:EGFP;myogkg128/+fish were incrossed and progeny imaged by confocal microscopy. Lateral and three equi-spaced transverse images of somite 17 were collected from each larva at each stage (dashed lines). Transverse area (red outline) multiplied by somite length (cyan dashed line) yielded myotome volume for each fish at each stage.eOptical transverse-sections ofβ-actin:EGFP;myogkg128mutants show reduced myotome area at 2, 3 and 5 dpf compared to sibs (dashed red lines). Boxes are shown magnified beneath highlighting smaller fibre cross-sections in mutants (dashed white lines). Representative imagesn= 6 mutants,n= 14 sibs (2 dpf);n= 5 mutants,n= 18 sibs (3 dpf);n= 9 mutants,n= 13 sibs (5 dpf).fMyotome volume reduction inmyogkg128mutants at 2, 3 and 5 dpf.g–i. Myotome length (g), number of fast fibres per cross section (h) and fibre volume (i) at 2 dpf compared byttests. Bars = 50 μm. nt: neural tube, nc: notochord 5a, b ), showing that other factors drive mymk expression in some cells. Residual mymk mRNA is preferentially enriched in the medial region of mutant myotome, adjacent to the notochord (Fig. 6a ). Notochord-derived Hedgehog (Hh) signals promote differentiation of slow and a medial subset of fast muscle in zebrafish [19] , [30] , [35] , [37] , [50] , [51] , [52] , [53] , [54] . Treatment of myog mutant embryos with the Hh inhibitor cyclopamine (CyA) led to an additional 54% reduction of mymk mRNA, leaving < 20% of the original mymk expression compared to vehicle-treated wt siblings (Fig. 6b ; Supplementary Fig. 5c,d ). CyA-treated sibs also showed a 22% mymk reduction (Supplementary Fig. 5c–e ) compared to controls. Congruently, when a β-actin:EGFP;myog kg125/+ incross was treated with CyA, residual fusion in myog mutants at 2 dpf was largely lost (Fig. 6c ). Blockade of Hh signalling had no detectable effect on fusion in sibs, although reducing both sib and mutant fast muscle growth, as previously reported [55] (Fig. 6c ). These observations show that in myog mutants Hh signalling sustains residual mymk expression and myocyte fusion in the deep/medial myotome close to the notochord. Fig. 6 Hedgehog signalling sustains residual fusion and mymk expression. a ISH for myomaker ( mymk ) at 20 hpf revealed that residual expression in myog mutant is enriched in the medial region of the somite close to notochord (arrows in transverse sections from indicated axial level, dorsal to top). Note lack of expression in mononucleate slow pioneer fibres (arrowheads, upper panel). Representative images n = 6 mutants, n = 14 wt sibs ( mymk ) b ISH (lateral view, dorsal to top) and qPCR analysis showing that cyclopamine (CyA) treatment of myog kg125 embryos almost abolished mymk mRNA compared to ethanol (EtOH) vehicle control. CyA effectiveness is shown by the absence of unstained slow muscle pioneer cells (arrowhead). Mean fold change ± SEM from three independent experiments on embryos from separate lays of myog kg125 (circles) and myog kg128 (squares and triangles) analysed on separate days, paired t test statistic. Representative images n = 4 EtOH, n = 6 CyA. c Optical confocal sections of the medial region of somites 17 of β-actin : EGFP ; myog kg128/+ incross treated with vehicle or CyA. Transverse-section panels show medial position (yellow lines) of respective longitudinal section for each condition. CyA abolished residual fusion in the medial myotome of mutant embryos (arrowheads) but did not detectably affect fusion in sibs. Note that the residual multinucleate fibres in myog kg125 mutant appear larger than adjacent mononucleate fibres in EtOH but are lacking in CyA. nt: neural tube, nc: notochord. Representative images n = 5 mutants, n = 3 sibs (EtOH); n = 4 mutants, n = 6 sibs (CyA). Bars = 50 μm Full size image Adult myog mutants have small muscle with reduced fibre size Both putative null myog alleles are homozygous viable. By 4 months (120 dpf), compared to their co-reared sibs, adult mutants showed a reduction in standard weight, a measure that compensates for length changes (Fig. 7a, b ; Supplementary Fig. 6a, b ). In contrast, myog fh265 mutants were similar to sibs, consistent with the lack of larval phenotype (Fig. 7b ; Supplementary Fig. 6a ). The new mutants showed a 35-40% reduction in weight and lower ‘body mass index’. These data show that muscle bulk reduction is independent of, and may cause, the observed length reduction (Supplementary Fig. 6a ). Muscle reduction persisted also in 15 month old mutants (Supplementary Fig. 6c ). Fig. 7 Adult Myogenin mutants have reduced muscle with more but smaller myofibres. a Myog mutant and sib at 120 dpf from myog kg128/+ incross. Bar = 1 cm. Representative images n = 5 mutants, n = 23 sibs. b Myog kg128 or myog kg125 but not myog f fh265 showed reduced standard weight compared to co-reared sibs at 120 dpf. Dots represent individuals. c Laminin immunodetection on cryosections from 120 dpf myog 128/+ incross. Bar = 100 µm. Representative images, n = 3. d – f Number of muscle fibres in 0.1 mm 2 of adult muscle is increased in mutants ( d ), whereas myofibre cross-sectional area (CSA) is decreased ( e ) reflecting a shift in CSA frequency distribution compared to sibs. g Fewer myonuclear profiles were present within laminin profiles in adult muscle cross-sections in mutants than in sibs, measured from 107 to 490 fibres at similar medio-lateral and dorso-ventral positions of trunk muscle of three fish per genotype. Mean ± SEM, t test. h Proportions of muscle fibres with indicated number of myonuclei within fibre cross-sectional profile. In sibs, >90% of fibres have more than one nuclear profile, compared with < 15% in mutants. Mean ± SEM, χ 2 test. i NADH tetrazolium reductase stain revealed that in both mutants and sibs three fibre types are present: oxidative/slow (slow), intermediate (int) and glycolytic/fast (fast). Size of more glycolytic myofibres (yellow and green insets) is more reduced than oxidative fibres (cyan). Assay was performed on three 120 dpf adult male length-matched fish of each genotype. Representative sib (blue) or mut (red) fibres are highlighted. Mutant presents smaller slow type myofibres ectopically localised in fast domain (red inset). Representative images, n = 3. Bars = 100 μm (except for red, yellow and cyan insets = 10 μm) Full size image Adult muscle phenotype examined in transverse cryosections of 120 dpf myog kg128 incross fish revealed a decreased myotome area, reduced fibre cross-sectional area and increase in fibre number per unit area of muscle in myog kg128 mutants, compared to matched sibs (Fig. 7 c–f; Supplementary Fig. 6b ). The total number of fibres in single body cross-sections of a mutant (4097) and a heterozygote sib (3657) were similar and were approximately 40-fold those in larvae, indicating that fibre formation had persisted (Supplementary Fig. 6b ). The number of nuclei in mutant fibre cross-sections was reduced threefold compared to sibs, but a few fibres with several nuclei were still present (Fig. 7g,h ; Supplementary Fig. 6d, e ). The total area of both slow and fast muscle also appeared reduced (Fig. 7i ; Supplementary Fig. 6b ). Fibre typing for oxidative metabolism revealed that fast muscle fibre size was more reduced than slow fibre size. 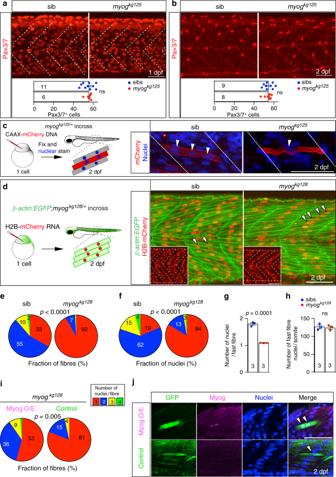Fig. 4 Myogenin promotes fusion of myocytes.a,bImmunodetection and quantification of Pax3/7 positive MPCs in somite 17 ofmyogkg125/+incross embryos at 1 dpf and 2 dpf. Mean ± SEM of dots representing individual embryos. Lack of Myog does not alter number of Pax3/7 MPCs per somite (white dashed lines). Representative imagesn= 6 mutants,n= 11 sibs (1 dpf);n= 8 mutants,n= 9 sibs (2 dpf).cQualitative analysis of myoblast fusion in amyogkg125/+incross injected at 1-cell stage with DNA encoding CAAX-membrane targeted mCherry (red). At 2 dpf, larvae were fixed and stained with Hoechst to highlight nuclei (blue) and analysed from 3D stacks. Nuclei within mCherry-labelled fibres (arrowheads) were mostly single in mutants, but multiple in sibs. Representative imagesn= 6 embryos.dMyoblast fusion quantified by injection ofH2B:mCherryRNA into 1-cell stage embryos fromβ-actin:EGFP;myogkg128/+incross. Confocal single plane images deep in the myotome of 2 dpf larvae showing muscle fibres and the position of nuclei (insets). Note the central location away from somite borders (dashed white lines) of most nuclei in mutants (arrowheads), similar to that observed in mononucleate superficial slow fibres. Representative imagesn= 6 embryos.e,fQuantification of fusion within the entire myotome 17, showing the fraction of fast fibres (e) and fraction of nuclei in fast fibres (f) with the indicated number of nuclei. Slow fibre numbers were unaltered. Data report mean values of three larvae per genotype (see Supplementary Fig.3afor individual data).p-values indicate probability of rejecting null hypothesis of no difference between mutant and sibs inχ2tests.gNumber of nuclei per fast fibre is reduced in mutant.hTotal number of nuclei within fast fibres in somite 17 of sib and mutant is unchanged. Dots represent individual embryos. Mean ± SEM.ttest. Bars = 50 μm.i,jMosaicmyog:MyogCDS-IRES-GFPplasmid-derived expression of Myog (Myog O/E) rescues fusion inmyogkg128mutant larvae from amyogkg128/+incross, compared controlmyog:GFPplasmid (Control). Quantification (as ine) of nuclei in GFP+cells (i, see Supplementary Fig.4afor individual data). Immunodetection shows Myog overexpression (Myog O/E, magenta) inmyog:MyogCDS-IRES-GFPbut not inmyog:GFP(Control, green) GFP+fibres (j). Representative imagesn= 5myog:GFP,n= 11myog:MyogCDS-IRES-GFPinjected mutants, ns: not significant Interestingly, the slow muscle region overall appeared less oxidative and fibres in the intermediate and slow regions were disorganised and smaller in mutant fish (Fig. 7i ). Thus, fish lacking Myogenin have severe defects in adult muscle. Fusion defect in adult-derived myog mutant MPCs To determine whether the deficits in mutant adults derived from defective development alone, or persisted due to a Myog requirement in the adult, we analysed cellular dynamics of adult-derived muscle progenitors cells (MPCs) ex vivo. Initially, we developed a method to culture satellite cells derived from isolated fibres of adult zebrafish that yielded MPCs that could undergo terminal differentiation, up-regulate desmin and accumulate MyHC and fuse into myotubes in vitro (Fig. 8a ). Strikingly, myog mutant MPCs differentiated as well as sibling MPCs (Fig. 8b ), but showed a dramatic reduction in cell fusion compared to heterozygote controls (Fig. 8a–d ). Indeed, fusion index declined greatly; whereas the majority of sibling myotubes contained three or more nuclei, 98% of mutant myotubes were mononucleate (Fig. 8c, d , Supplementary Fig. 6f ). Differentiating Myog-deficient MPCs expressed desmin and MyHC, elongated and aligned similarly to control cells (Fig. 8a, b ; Supplementary Fig. 6g ). These data show Myog is not required for terminal differentiation of satellite cell-derived MPCs into myocytes but is required for myocyte fusion throughout life. Fig. 8 Mutant adult-derived muscle progenitor cells retain fusion deficit ex vivo. a Immunodetection of desmin (green) and MyHC (red) and nuclei (white, Hoechst) in 15 months old myog kg125 and sibling myog kg125/+ adult-derived MPCs following 5 days of differentiation. Fusion into multinucleated myofibres occurred only in sib (magnified boxes), coloured arrowheads indicate nuclei of each cell. Representative images, n = 3. b Extent of differentiation (Differentiation index) is comparable between mutant and heterozygous MPCs. c Fusion index showing deficit in fusion of mutant myocytes. d Number of nuclei in fused MyHC + cells is reduced in mutant, χ 2 test. Three fish per genotype (three technical replicates each). e Schematic of the role of Myogenin during differentiation, fusion and growth of muscle fibres. During myogenesis, committed MPCs leave the cell cycle, begin to elongate and express early muscle-specific genes during terminal differentiation into myocytes. At this stage, Myogenin (MYOG) promotes the expression of myomaker (MYMK), myomixer (MYMX) and jam3b (JAM3B). These fusogenic proteins prompt myocyte fusion to form muscle fibres. In the absence of Myogenin, myocytes undergo terminal differentiation but fail to express Myog-module genes, remain mononucleated and grow less throughout life. Residual myocyte fusion in Myog mutants in the medial region of the somite (bracket) is sustained by Hedgehog (Hh) signalling Full size image The data presented radically change the interpretation of the evolutionarily conserved role of Myog in skeletal muscle development through four major findings. First, Myog is not required for terminal differentiation of most myoblasts into myocytes. Second, Myog has a major conserved role in driving the fusion of myocytes into multinucleate fibres. Third, that a second, Myog-independent, pathway to muscle fusion exists and, in the zebrafish trunk, is promoted by Hh signalling. Lastly, that Myog is required for normal myogenesis throughout life and that its loss leads to poor muscle and whole body growth and a persistent functional fusion deficit in adult satellite cell-derived muscle progenitors. In mice lacking Myog, myoblasts can form myocytes expressing proteins of the contractile apparatus [5] , [6] , [7] , [8] . However, a major deficit of early muscle formation was reported, with dramatic downregulation of MyHC at e12.5 in both trunk and limb muscle and a worsening deficit in neonates [7] , [8] . This led to the view [2] , that ‘Myogenin knockout has a …. complete absence of functional skeletal muscle’. Our data from zebrafish contradict this view; we observe differentiated muscle fibres, normal sarcomere formation and normal numbers of nuclei within fibres in the larval myotome of mutants. Nevertheless, although to our knowledge no compelling images of fusion in the absence of Myog in vivo have been published, cultured myoblasts and satellite cells from Myog mutant mice are reported to fuse and myocytes lacking Myog can fuse with wild-type myocytes in vivo in murine chimaeras [7] , [11] . We conclude that Myog is dispensable for terminal differentiation of myoblasts into post-mitotic myocytes and contractile myofibres in zebrafish (Fig. 8e ). Early reports suggested that murine myotomal Myog protein does not accumulate until after muscle differentiation, despite the earlier presence of Myog mRNA [56] , [57] . Moreover, embryonic MyHC ( Myh3 ) mRNA is almost normally expressed in e14.5 Myog mutants, whereas maturation to expression of perinatal MyHC ( Myh8 ) mRNA is dramatically reduced at e18.5 [7] , [8] . The widespread accumulation of desmin protein, hitherto taken as an indication of a myoblast state [7] , [8] , [58] , could instead reflect myocyte formation. The ability of myogenic cells from Myog −/− to form myotubes in culture also argues for unimpaired myocyte formation [6] , [7] . Consistent with murine data [8] , we find that balance of zebrafish slow and fast fibre formation is unaffected by loss of Myog. However, our finding that several genes required for later steps in myocyte differentiation (e.g. fusion) are down-regulated in mutants indicates that a subset of muscle differentiation genes, the ‘Myog-module’ are regulated by Myog in zebrafish (Fig. 8e ). Zebrafish Myog is not essential for, but can promote, muscle terminal differentiation. We previously reported that loss of both Myf5 and Myod ablates all skeletal myogenesis, whereas combined reduction of Myod and Myog severely reduces fast muscle [17] , [18] . These findings show that, in the absence of MyoD, Myf5 requires Myog to drive fast myogenesis [17] . Interestingly, even hypomorphic myog fh265 mutants that lack a developmental fusion defect show poor muscle regeneration and apoptosis of myf5 -marked cells [20] . Hence, we cannot exclude the possibility that a non-essential subset of myoblasts requires Myog for terminal differentiation in older zebrafish. Lack of Myog is not compensated by increased expression of myod and leads to downregulation of mrf4 mRNA, as observed in mice lacking Myog [5] , [7] , [8] , [12] . Surprisingly, we found that myog mutant embryos accumulate less myf5 mRNA, suggesting that Myog may promote myf5 expression or be required for the production of myf5 -expressing cells. Myog mutants have a severe lack of fusion, despite efficient myocyte differentiation. We find that myog activity is essential for normal expression of a subset of fusogenic genes, mymk, mymx and jam3b , mutation of which causes fusion defects strikingly similar to the myog mutant phenotype [23] , [24] , [25] , [48] , [49] , [59] . We propose, therefore, that early terminally-differentiated fast myocytes are primed for fusion, but lack sufficient expression of critical Myog-module components until Myog becomes active (Fig. 8e ). Interestingly , mymk mRNA was more highly reduced than any other gene analysed, which could account for the fusion defect observed. However, as jam3b mRNA is more widely expressed [48] , [60] , its lesser reduction may reflect strong reduction in muscle and unaltered expression elsewhere. Thus, the extent of the Myog-module functionally required for fusion remains to be determined. Mosaic Myog re-expression in myog mutant fully rescues fusion. Strikingly, this effect is cell autonomous and fairly efficient, which leads to several important conclusions. Firstly, as two adjacent GFP-marked cells are rare, a single isolated Myog-expressing myocyte appears sufficient to induce fusion to an adjacent cell lacking Myog. This result parallels the chimaera analysis showing fusion of Myog −/− with wild-type cells in murine myogenesis [11] . Secondly, the existence of rescued fibres with more than two nuclei suggests that Myog expression in a binucleate fibre can elicit fusion of adjacent cells lacking Myog. It may be significant in this regard that Jam3b, Mymk and Minion/Myomerger/Myomixer have been shown to be required in only one cell of a fusing pair, although fusion efficiency was reportedly higher when both cells express Mymk [24] , [47] , [48] . We observed that Myog occupies E-boxes in the endogenous mymk 5' proximal region during the period of fusion in vivo. A 3 kb mymk promoter fragment containing these sites drives reporter expression in zebrafish fast muscle [24] . Similarly, in mouse and chick, Mymk expression parallels that of Myog and depends on conserved E-boxes, including one at -41 bp [61] , [62] . Moreover, in cultured myocytes, Myog binds to conserved sequences in Mymk, Mymx and Jam3 ( www.encodeproject.org/experiments/ENCSR000AID ). Interestingly, the early Xenopus, chick and mouse myotomes are reported to be composed of mononucleate fibres [63] , [64] , [65] , [66] , [67] . As the murine Myog mutant shows little early defect, but even partial deletion of a floxed Myog allele after initial fibre formation shows that Myog is essential for late embryonic and neonatal myogenesis [12] , [13] , the data on murine Myog mutants are all consistent with a primary fusion defect. Moreover, some reports in C2C12 cells have suggested that Myog expression correlates with, and is required for, myocyte fusion, although conflicting findings exist [68] , [69] . We note that zebrafish slow muscle fibres, which remain mononucleate long after their terminal differentiation, accumulate much lower levels of myog mRNA than fast muscle precursors, paralleling their lower levels of mymk and mymx mRNA [17] , [18] , [19] , [59] , [70] . However, although overexpression of Myog in slow myocytes reduces their size and alters myofibril organisation, it did not drive their fusion to each other or to adjacent fast myocytes, in contrast to mymk overexpression [24] . Zebrafish myog mutants show a similar increase in number of myofibres to that reported when fusion is blocked in mutants lacking Jam proteins [48] . In the case of myog mutants, the increase in fibres was quantitative; total nuclear number in myofibres remained constant, suggesting that normal numbers of myoblasts differentiated, survived and made fibres. It seems that during early myotome formation, therefore, either no specific sub-population of ‘founder’ myoblasts determines fibre number, as occurs in Drosophila embryonic myogenesis [71] , [72] or Myog is required to prevent cells acting as founder cells. Interestingly, previous studies reported that fusion-defective myoblasts elongate and differentiate into mononucleated muscle fibres [23] , [24] , [48] , [49] . We hypothesise that, like fish, murine Myog mutants are blocked in fusion. Perhaps lack of fusion triggers loss of nascent myocytes that fail to form attachments to skeleton or nerve. In addition, myoblast populations such as those in neonatal limb may absolutely require Myog for terminal differentiation. In myog mutant fish a small group of muscle fibres in the deep myotome undergoes fusion. Residual fusion was also observed in jam3b and jam2a mutants and mymk mutants were also stated to be only ‘predominantly mononucleated’, although the extent and location of residual multinucleate fibres was not reported [24] , [48] . We find that Myog-independent fusion requires Hh signalling, probably from adjacent midline tissue, which also up-regulates mymk mRNA in the deep myotome. The low residual level of mymk mRNA observed in CyA-treated myog mutants could reflect incomplete loss of Hh function, or additional controls on mymk expression. As Hh promotes slow and fast muscle differentiation through activation of Myod by a Cdkn1c/p57 positive feedback loop [19] , we speculate that Hh-induced fusion may arise from increase in Myod-driven mymk expression in myocytes adjacent to the midline source of Hh. Our data suggest that distinct myocyte fusion processes contribute to muscle fibre diversity. Our study quantified the extent of fusion in wild-type and myog mutant fast muscle. Interestingly, a significant minority (~30%) of fast fibres are mononucleated at 2 dpf in wild-type, meaning that ~20% of fast myocytes had not yet fused. Many of these may reflect dermomyotome-derived fast myocytes that had recently undergone terminal differentiation, because they were predominantly located in the lateral myotome [36] , [38] . Nevertheless, transplant experiments have reported rates of fusion above 95% [24] , [48] , implying that a rare subset of proliferative somite cells generates the mononucleate fast fibres. On the other hand, in myog mutants only about 20% of myocytes fuse. As frequencies of residual fusion are yet to be reported in jam2a , jam3b , mymk and mymx mutants [23] , [24] , [48] , [59] , it is unclear whether some fusion mutants have more severe defects than others. Myog mutants are viable but grow less rapidly than their sibs. Early in life, myog mutants have small fibres and reduced myotome size, which might give them a disadvantage in competitive feeding leading to reduced growth. Alternatively, Myog could be required for some other function, such as synthesis of myokines important to coordinate whole body scaling of tissue size. However, adult mutants have a disproportionate loss of muscle compared to their length and a persistent greatly reduced fibre size and nuclear content throughout life that could reflect defective adult MPC differentiation. Zebrafish muscle has been shown to contain fibre-associated satellite cells [41] , [73] , [74] . To address the role of Myog in adult life, we developed an MPC culture procedure for zebrafish satellite cells. This method shows that adult MPCs lacking Myog undergo terminal differentiation but fuse poorly ex vivo, indicating that Myog is required throughout life, rather than that the defect in adult fish derives solely from persistence of early developmental defects that are subsequently Myog-independent. Definitive proof of this conclusion will require deletion of myog function in adult fish. Nevertheless, combined with the defective regeneration of larval muscle in myog hypermorphs [20] , our data strongly suggest that Myog also functions during adult muscle growth and regeneration. In striking contrast to the myog mutant phenotype, lack of Myod reduces fibre number in larvae without affecting fusion or mymk expression, and the remaining fibres grow larger [45] . In myod mutants, a reduction in the number of fast fibres is accompanied by an increase in MPCs expressing Pax3 and/or Pax7, presumably reflecting reduced terminal differentiation [18] , [45] . Given that Myod can activate myog expression and either MRF can drive terminal differentiation of fast fibres [17] , these opposite effects on fibre number and size suggest that the balance of MRFs influences the mode of muscle growth. Several studies in mice have also implicated MRFs in adult fibre size control [14] , [75] , [76] . Like zebrafish, mice conditionally lacking Myog in the adult show reduced body and fibre size, although nucleation state of mutant myofibres was not reported [12] , [13] , [14] . However, in contrast to its role in promoting fusion and fibre growth in developing muscle, in the adult context Myog appears to promote fibre atrophy upon denervation and regulate metabolic capacity in innervated muscle [14] , [77] . Moreover, Myog overexpression in both multinucleate fast muscle in mice and, as shown here, in mononucleate slow fibres in larval zebrafish leads to reduced fibre diameter [75] . As suggested by the differences in Myog-regulated genes in embryonic and adult cells [13] , it seems that Myog performs distinct functions in myoblasts, nascent myocytes and mature fibres. Zebrafish lines and maintenance All lines used were reared at King’s College London on a 14/10 h light/dark cycle at 28.5 °C with adults kept at 26.5 °C, with staging and husbandry as described [78] . 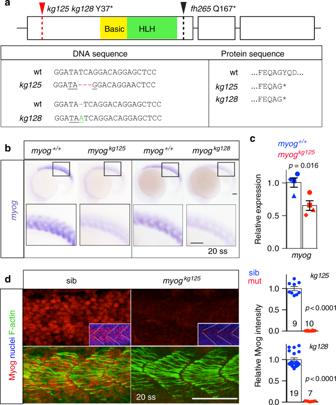Embryos/larvae were reared at 28.5 °C in the dark, except for periods outside the incubator. myog fh265 and myod fh261 mutant alleles [18] , [45] on AB background were genotyped by sequencing as described previously [18] . 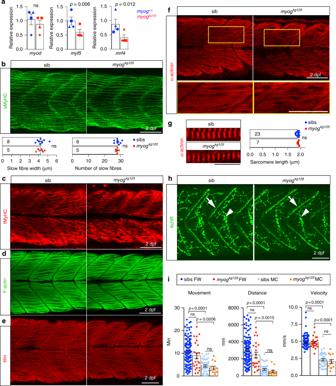Fig. 1 Genome editing generates zebrafishmyognull alleles.aSchematic ofmyoggene exons (boxes) and protein showing the position ofkg125,kg128andfh265mutant alleles. The tyrosine to stop mutations (Y37*) produce a truncated protein of 36 amino acids (aa) devoid of both basic (yellow) and helix–loop–helix (HLH, green) domains. Thefh265hypomorphic allele (Q167*) truncates downstream of bHLH. Beneath, DNA and protein alignment of wild-type (wt), 3 bpkg125deletion (red) and 1 bpkg128insertion (green) alleles with novel stop codons underlined causing an identical truncation.bIn situ mRNA hybridisation (ISH) formyogeninonmyogkg128/+andmyogkg125/+incross lays reveal NMD of mutantmyogmRNA at 20 somite stage (20 ss). Representative imagesn= 14 + 5 mutants,n= 39 + 22 sibs, respectively. Insets show magnification of boxed areas.cqPCR analysis on wt sibs andmyogkg125embryos at 22 ss confirms NMD. Mean fold change ± SEM from four independent experiments on genotyped embryos from four separate lays analysed on separate days, pairedttest statistic. Symbol shapes denote matched wt and mutant samples from each experiment.dImmunoreactivity of Myog is lost inmyogkg125andmyogkg128mutants at 20 ss, whereas F-actin is unaffected. Insets show nuclear staining inmyogkg125and sib using Hoechst counterstain. Relative myotomal Myog immunofluorescence was assessed by nuclear intensity measurement. All images are lateral views anterior to left, dorsal to top. Representative imagesn= 10 + 7 mutants,n= 9 + 19 sibs, respectively. Bars = 50 µm myog kg125 and myog kg128 , on the TL background, were genotyped by sequencing or by loss of EcoRV site in the mutant alleles, following PCR amplification using primers indicated (Supplementary Table 1 ). Fig. 2 Functional muscle differentiation in Myogenin mutants.aqPCR analysis on wt sibs andmyogkg125embryos at 22 ss showing reduction ofmyf5,mrf4but notmyodRNAs. Mean fold change ± SEM from four independent experiments on genotyped embryos from four separate lays analysed on separate days, pairedttest statistic. Symbol shapes denote matched wt andmyogmutant samples from each experiment.b,cImmunodetection of slow and fast myosins (sMyHC and fMyHC) in 2 dpf larvae from amyogkg125/+incross showing that myofibre differentiation occurs in mutant. Dots in graphs show slow myofibre width (average of six myofibres/larva) and number in somite 17 of sib and mutant individuals. Representative imagesn= 5 mutants,n= 8 sibs.d–fPhalloidin staining for F-actin or immunolabelling for titin and α-actinin reveals that mutant myofibres display regular sarcomere spacing and are properly assembled to sustain contraction. Representative imagesn= 5 mutants,n= 21 sibs (phalloidin);n= 7 mutants,n= 18 sibs (titin);n= 7 mutants,n= 23 sibs (α-actinin). Inf, boxes are shown magnified below.gSarcomere length fromf(average of 6 myofibres/larva) in sibs and mutants. Numbers of larvae analysed are shown on columns (b,g).hLarvae from amyogkg128/+incross stained with α-bungarotoxin-Alexa-488 show that mutant embryos accumulate AChR at both neuromuscular junction (arrows) and muscle-muscle junction (arrowheads) comparable to sibs. Representative imagesn= 4 mutants,n= 11 sibs.iMotor function of 5 dpf larval zebrafish in fish-water (FW;n= 24 mutants,n= 115 sibs) or 0.6% Methyl-Cellulose (MC;n= 12 mutants,n= 36 sibs) as time spent moving (minutes), distance travelled (mm) and average speed (mm/s). Overall muscle function is unaffected by lack of Myog in both FW and MC. Activity of bothmyogmutants and sibs is affected by MC. Each dot represents the behaviour of an individual larva. ns: not statistically significant in ANOVA. Bars = 50 µm (10 µm ing) The two new alleles had indistinguishable phenotypes and no differences were detected between wt and heterozygous fish, so we refer to mutants and siblings (sibs), and report the specific myog allele in each experiment in Figures and Supplementary Table 2 . Tg(Ola.Actb:Hsa.HRAS-EGFP) vu119 (ref. [33] ) was originally on King’s wild-type background. All experiments were performed on zebrafish derived from F2 or later filial generations, in accordance with licences held under the UK Animals (Scientific Procedures) Act 1986 and later modifications and conforming to all relevant guidelines and regulations. Embryo manipulation Myogenin mutants were generated targeting the sequence 5′-GGAGCTCCTGTCCTGATATC-3′ on the reverse strand using CRISPR/Cas9 method as previously described [79] . Mutant lines, myog kg125 and myog kg128 , were bred onto Tg(Ola.Actb:Hsa.HRAS-EGFP) vu119 . Muscle (myotome) size was analysed as previously described [18] , [45] and schematised in Fig. 3d , except for myog fh265/+ incross embryos, which were immersed in 3 μM BODIPY-FL-C5 (Thermo Fisher Scientific) in fish water (FW) from 30 hpf until 2 dpf, washed twice and agarose-mounted for live imaging [18] , [45] . H2B-mCherry capped RNA (100 pg per embryo, kind gift from H. Roehl, University of Sheffield, UK and S. Megason, Harvard Medical School, USA) or DNA plasmid encoding membrane targeted CAAX-mCherry (25 pg per embryo [80] ) were injected into 1- to 2-cell stage embryos to analyse fusion. Morpholino antisense oligonucleotide against myog [17] , [18] (2 ng per embryo) was injected into 1- to 2-cell stage Tg(Ola.Actb:Hsa.HRAS-EGFP) vu119 embryos, which were fixed with 4% paraformaldehyde (PFA) for 15 min, at 20 ss when knockdown efficiency was checked by Myog immunodetection, or at 2 dpf and incubated overnight with Hoechst 33342 (Life Technologies). Cyclopamine [81] (50 μM) or ethanol vehicle control was added at 50% epiboly to embryos with chorions punctured with fine forceps. Motor function was assayed at 5 dpf in a 30 min trial using DanioVision (Noldus) and EthoVision XT9 tracking software. Larvae were acclimatised in 0.6% methyl-cellulose (MC, Sigma Aldrich) or FW vehicle control in 24-well plates for at least 2 h before tracking. Following tracking, larvae were raised in MC or FW and analysed by confocal imaging at 8 dpf. Rescue assay Myogenin coding sequence was PCR amplified from pBluescript SK-MG12-ZF -Myogenin [70] using listed primers (Supplementary Table 1 ) and subsequently cloned into hsp70-4:MyogCDS-IRES-NLSmGFP6 [82] . MyogCDS-IRES-NLSmGFP6 insert was then PCR amplified from hsp70-4:Myog-IRES-NLSmGFP6 . myog promoter:GFP vector ( myog:GFP ) [83] was linearised by PCR removing GFP sequence using listed primers (Supplementary Table 1 ). Final myog:MyogCDS-IRES-GFP plasmid was made using Gibson Assembly (E2621, NEB) and sequence verified (Genbank:MH593821). Rescue experiments were performed by injecting 20 pg myog:MyogCDS-IRES-GFP or myog:GFP control into 1- to 2-cell stage myog kg128/+ incross lays. Embryos were fixed at 2 dpf and processed for immunostaining for Myog, GFP, slow MyHC (F59) and Hoechst 33342 as described below. Each embryo was then mounted for confocal scanning of somites 15-20 on one side and nuclei within GFP + fibres were counted. Imaging and in situ mRNA hybridisation and immunodetection ISH and immunodetection were performed as described [84] . Briefly, fish were fixed in 4% PFA in phosphate-buffered saline (PBS) for 30 min or 3 h at room temperature or overnight at 4 °C. Embryos for ISH were stored in 100 % methanol at −20 °C and rehydrated in PBS prior to ISH. Fish for immunostaining were permeabilised in PBS 0.5% Triton X-100 (PBSTx) for 5 min, blocked in Goat Serum 5% (Sigma Aldrich) in PBSTx and incubated with primary antibodies at indicated concentrations at least overnight. Fish were then washed in numerous changes of PBSTx for at least 5 min and incubated and washed similarly with indicated secondary antibodies and prepared for imaging as described below. Primary antibodies against Myog (M-225 Santa Cruz Biotechnology, 1:50), fast MyHC (EB165 (1:2), Developmental Studies Hybridoma Bank, Iowa (DSHB)), slow MyHC (S58 (1:2) or F59 (1:5), DSHB) or MyHC (A4.1025 (1:5) [30] , MF20 (1:300, DSHB)), α-actinin (1:500, A7732, Sigma Aldrich), Pax3/7 (DP312 (1:50), Nipam Patel, UC Berkeley, USA), Laminin (L9393 (1:400), Sigma Aldrich), GFP (13970 (1:400), Abcam), Titin (T12 (1:10), D. Fürst, University of Bonn, Germany), desmin (D8281 (1:100), Sigma Aldrich) were detected with Alexa-conjugated secondary antibodies (Invitrogen) and Goat anti-Mouse IgA-FITC (Serotec). Digoxigenin-labelled probes were against myog [70] , smyhc1 [27] , mylpfa [26] or mymk , jam3b , jam2a and kirrel3l made by PCR on 1 dpf cDNA template using listed primer pairs (Supplementary Table 1 ) with an added T7 polymerase binding site. For confocal imaging, embryos were mounted in glycerol, Citifluor (Agar) or 0.8–1% low melting point agarose and data collected on the somites 17-18 near the anal vent on a LSM Exciter microscope (Zeiss) equipped with 20 × /1.0 W objective and subsequently processed using either Volocity (Perkin Elmer), Fiji (NIH, www.Fiji.sc ) or ZEN (Zeiss) software. 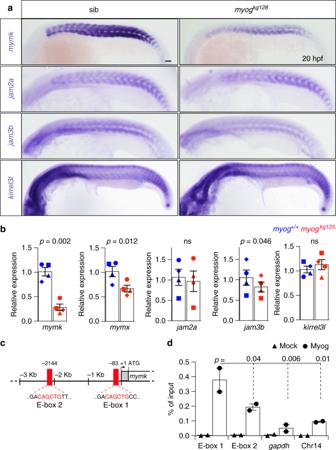Fig. 5 Myogenin mutants have reduced expression of fusogenic factors.aISH on 20 hpfmyogkg128/+incross to investigate the expression of genes essential for vertebrate myocyte fusion. Expression ofmyomaker(mymk) andjam3b, but not ofjam2aorkirrel3l, is reduced inmyogmutant. Bar = 50 μm. Representative imagesn= 10 mutants,n= 38 sibs (mymk);n= 13 mutants,n= 37 sibs (jam2a);n= 12 mutants,n= 39 sibs (jam3b);n= 7 mutants,n= 13 sibs (kirrel3l).bqPCR analysis of RNA expression levels showing downregulation ofmymk,myomixer/myomerger/minion(mymx) andjam3bat 20 hpf onmyogkg125mutants, whereasjam2aandkirrel3lremain unaltered compared to wt (myog+/+) sibs. Graphs show mean fold change ± SEM of four independent experiments; pairedttest. Symbol shapes denote wt and mutant samples from paired experiments.cSchematic of 5' genomic region ofmymkreporting: 5′-UTR and coding sequence (grey and white boxes), position of E-box elements (red boxes), relative bp distance from 5'UTR start (+1), start codon (arrow, ATG). E-box 1 and E-box 2 sequences are shown in red text.dChIP-qPCR assay using anti-Myog or mock showing significant Myogenin enrichment onmymkE-box 1 compared to negative controls from thegapdhpromoter and a gene-free region on chromosome 14 containing an E-box (Chr14). Mean of percentage of input immunoprecipitated ± SD of two independent experiments, ANOVA Myotome volume, number of fibres and fibre volume were calculated as described [45] and schematised in Fig. 3d . α-Bungarotoxin-Alexa 488 (Invitrogen) and phalloidin staining was as described [85] . Myogenin immunofluorescent intensity was averaged from at least 10 randomly-selected nuclei at similar dorso-ventral and mediolateral position within somites 9-10 of each embryo. Nuclei of interest (NOI) were selected blind by Hoechst 33342 staining then Myogenin fluorescence was quantified in selected NOI using Fiji. To account for staining variability between embryos, background was subtracted from nuclear Myogenin intensity in each embryo by measuring fluorescence intensity of nucleus-free areas of an equal size to the NOI in each somite region (see Supplementary Fig. 1a for schematic). Relative average fluorescence intensity of nuclear Myogenin immunolabelling in mutant was then calculated relative to siblings. All images are shown as lateral views with anterior to left and dorsal up, unless otherwise stated. RT-PCR and qPCR myog kg125/+ incross embryos at 20 hpf were individually genotyped by sequencing using listed primers (Supplementary Table 1 ). RNA was extracted from pools of four embryos of each genotype using Trizol ® (Sigma Aldrich) and purified with RNA Clean & Concentrator™-25 (Zymo Research) or RNA Purification Plus Kit (Norgen). Total RNA (300 ng) was reverse transcribed using Superscript III reverse transcriptase (Invitrogen) following supplier’s instructions. qPCR on technical triplicates for each sample was performed on 5 ng of relative RNA using Takyon Low ROX SYBR 2X MasterMix blue dTTP (Takyon) on a ViiA™7 thermal cycler (Applied Biosystems). For each experimental sample, ΔCT was calculated by subtracting the CT value for housekeeping gene ( actb2 ) from that of the target gene. ΔΔCT of each target gene was then calculated by subtracting the average of the ΔCT obtained in the wt (sibilngs) samples from ΔCT for each sample. Relative gene expression was calculated using the 2 -ΔΔCT formula [86] and the fold change of the expression levels between sibs and mutants were compared using paired Student’s t test. Results are presented as mean ± SEM of fold changes from three or four independent experiments. Primers were purchased from Sigma-Aldrich (KiCqStart ® SYBR ® Green Primers Predesigned, Sigma Aldrich). All PCRs for genotyping and probe synthesis were performed using Phusion Taq polymerase (Life Technologies) on a T100 thermal cycler (Bio-Rad). Chromatin Immunoprecipitation and E-box enrichment analysis 3 Kb of putative promoter region of myomaker , retrieved from UCSC genome browser (GRCz10/danRer10), was scanned for E-box elements using JASPAR 2016 version (JASPAR CORE Vertebrata, jaspar.genereg.net) with default settings. To avoid false positive scoring, relative profile score threshold was set at 95-99%. 500–600 20 hpf wt TL embryos were processed as described [87] . For immunoprecipitation, 30 µg of chromatin were incubated with 4 µg of Myogenin antibody or normal rabbit serum as mock. 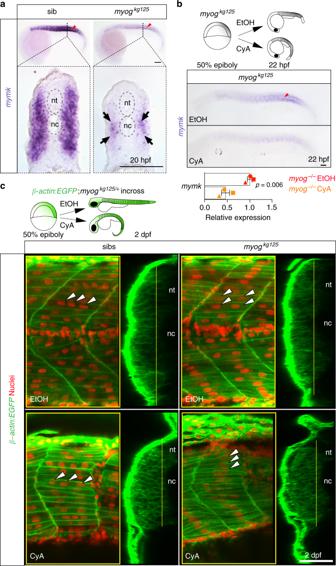Fig. 6 Hedgehog signalling sustains residual fusion andmymkexpression.aISH formyomaker(mymk) at 20 hpf revealed that residual expression inmyogmutant is enriched in the medial region of the somite close to notochord (arrows in transverse sections from indicated axial level, dorsal to top). Note lack of expression in mononucleate slow pioneer fibres (arrowheads, upper panel). Representative imagesn= 6 mutants,n= 14 wt sibs (mymk)bISH (lateral view, dorsal to top) and qPCR analysis showing that cyclopamine (CyA) treatment ofmyogkg125embryos almost abolishedmymkmRNA compared to ethanol (EtOH) vehicle control. CyA effectiveness is shown by the absence of unstained slow muscle pioneer cells (arrowhead). Mean fold change ± SEM from three independent experiments on embryos from separate lays ofmyogkg125(circles) andmyogkg128(squares and triangles) analysed on separate days, pairedttest statistic. Representative imagesn= 4 EtOH,n= 6 CyA.cOptical confocal sections of the medial region of somites 17 ofβ-actin:EGFP;myogkg128/+incross treated with vehicle or CyA. Transverse-section panels show medial position (yellow lines) of respective longitudinal section for each condition. CyA abolished residual fusion in the medial myotome of mutant embryos (arrowheads) but did not detectably affect fusion in sibs. Note that the residual multinucleate fibres inmyogkg125mutant appear larger than adjacent mononucleate fibres in EtOH but are lacking in CyA. nt: neural tube, nc: notochord. Representative imagesn= 5 mutants, n = 3 sibs (EtOH);n= 4 mutants,n= 6 sibs (CyA). Bars = 50 μm After purification of the immunoprecipitated DNA, enrichment was analysed by qPCR using primers listed in Supplementary Table 1 . Control primer pairs for genomic gapdh sequence and for chromosome 14 gene-free region were described [87] , [88] . All signals were normalised for input by percentage input calculation method ( www.thermofisher.com ). Adult fish analysis Siblings (120 dpf or 15 mpf) from heterozygote incrosses were anaesthetised with tricaine (Sigma Aldrich), blotted dry, weighed on an Ohaus YA102 balance, nose-to-base of tailfin length measured with a ruler and fin-clipped for sequence genotyping. Standard weight ( K ) was calculated using Fulton’s formula K = weight (g) × 100 × length −3 (cm)(reviewed in ref. [89] ). Body mass index (BMI) was calculated as ‘weight (g) × length −2 (cm)’. Three 120 dpf adult male length-matched fish of each genotype were culled using high dose tricaine, eviscerated and skinned. Trunk from just behind gills to 5 mm beyond the dorsal fin was embedded in OCT (CellPath, Fisher Scientific), immersed in freezing isopentane (Fisher Scientific) and stored at −80 °C. Cryosections (15 µm) from three anteroposterior positions were immunolabelled for Laminin and counterstained with Hoechst 33342 as described [90] and three or four images in consistent mediolateral and dorso-ventral somitic areas of sibs and mutants were acquired using an Axiovert 200 M microscope (Zeiss) equipped with LD A-plan ×20/0.85 objective. Fibre cross-sectional area (CSA) was measured in each image and averaged. Nuclei/fibre were scored as nuclei within laminin rings at three trunk positions in three fish of each genotype. The data are presented as the mean of averaged values from each individual fish. For digital whole section reconstruction several images where taken on iRiS™ Digital Cell Imaging System, using ×4 objective, and merged using Photoshop CS5.1. NADH Tetrazolium Reductase NADH-TR protocol was adapted from ( https://neuromuscular.wustl.edu/pathol/histol/nadh.htm ). Briefly, 15 µm unfixed cryosections, from three 120 dpf adult male length-matched fish of each genotype, were incubated in a 1:1 solution of NBT (Nitro-blue tetrazolium, 2 mg/ml, N6876, Sigma) and NADH (1.6 mg/ml, N8129, Sigma) in 0.05 M Tris HCl pH 7.6 at RT for 2 h. Sections were then washed three times with deionized water (dH 2 0), serially immersed in acetone:water 30%, 60%, 90%, 60%, 30%, ×3 dH 2 0, glycerol mounted and imaged with Axiophot microscope (Zeiss) equipped with Olympus DP-70 camera. Isolation and culture of zebrafish MPCs from adult tissue Isolation and culture of zebrafish adult muscle fibres was adapted from ref. [91] . Briefly, adult fish were culled in high dose tricaine, washed in PBS, then 70% ethanol, eviscerated and skinned. Trunk muscle was incubated in 0.2% Collagenase (C0130, Sigma Aldrich), 1% Penicillin/Streptomycin DMEM at 28.5 °C for at least 2 h. Single muscle fibres were released by trituration using heat-polished glass pipettes and washed three times with DMEM. 90–100 myofibres per fish were plated on Matrigel (Invitrogen) coated 24-well plates and cultured in 20% Foetal Bovine Serum in 1% Penicillin/Streptomycin/ DMEM for 7 days. Cells were washed twice with PBS to remove muscle fibres and induced to differentiate in 2% Horse Serum 1% Penicillin/Streptomycin/ DMEM for 5 days at 28.5 °C in 5% CO 2 with medium change every 48 h, then fixed with 4% PFA, processed for immunofluorescence and imaged at 20X using an Axiovert 200 M microscope (Zeiss). At least five random fields were acquired in each of three technical replicates on each fish. Six 15 months old adult male (three myog kg125/+ heterozygotes and three myog kg125 mutants) were dissected for the analysis. Differentiation index = nuclei in MyHC + myocytes (MF20 and A4.1025) × 100/nuclei in desmin + cells. Fusion index = Nuclei in myocytes with ≥ 2 nuclei × 100/ total nuclei in MyHC + myocytes. Statistical analyses Quantitative analysis on images was performed with Fiji software (NIH, Fiji.sc). 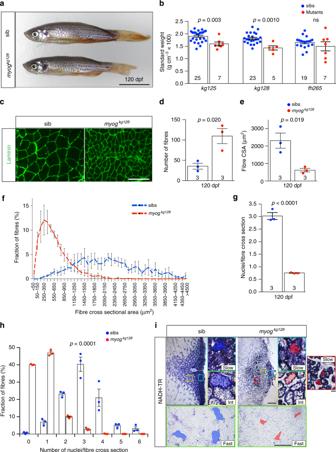Fig. 7 Adult Myogenin mutants have reduced muscle with more but smaller myofibres.aMyogmutant and sib at 120 dpf frommyogkg128/+incross. Bar = 1 cm. Representative images n = 5 mutants,n= 23 sibs.bMyogkg128ormyogkg125but notmyogffh265showed reduced standard weight compared to co-reared sibs at 120 dpf. Dots represent individuals.cLaminin immunodetection on cryosections from 120 dpfmyog128/+incross. Bar = 100 µm. Representative images,n= 3.d–fNumber of muscle fibres in 0.1 mm2of adult muscle is increased in mutants (d), whereas myofibre cross-sectional area (CSA) is decreased (e) reflecting a shift in CSA frequency distribution compared to sibs.gFewer myonuclear profiles were present within laminin profiles in adult muscle cross-sections in mutants than in sibs, measured from 107 to 490 fibres at similar medio-lateral and dorso-ventral positions of trunk muscle of three fish per genotype. Mean ± SEM,ttest.hProportions of muscle fibres with indicated number of myonuclei within fibre cross-sectional profile. In sibs, >90% of fibres have more than one nuclear profile, compared with < 15% in mutants. Mean ± SEM,χ2test.iNADH tetrazolium reductase stain revealed that in both mutants and sibs three fibre types are present: oxidative/slow (slow), intermediate (int) and glycolytic/fast (fast). Size of more glycolytic myofibres (yellow and green insets) is more reduced than oxidative fibres (cyan). Assay was performed on three 120 dpf adult male length-matched fish of each genotype. Representative sib (blue) or mut (red) fibres are highlighted. Mutant presents smaller slow type myofibres ectopically localised in fast domain (red inset). Representative images,n= 3. Bars = 100 μm (except for red, yellow and cyan insets = 10 μm) 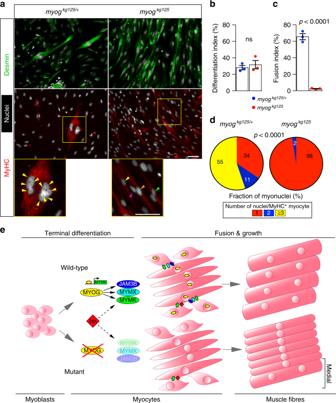Fig. 8 Mutant adult-derived muscle progenitor cells retain fusion deficit ex vivo.aImmunodetection of desmin (green) and MyHC (red) and nuclei (white, Hoechst) in 15 months oldmyogkg125and siblingmyogkg125/+adult-derived MPCs following 5 days of differentiation. Fusion into multinucleated myofibres occurred only in sib (magnified boxes), coloured arrowheads indicate nuclei of each cell. Representative images,n= 3.bExtent of differentiation (Differentiation index) is comparable between mutant and heterozygous MPCs.cFusion index showing deficit in fusion of mutant myocytes.dNumber of nuclei in fused MyHC+cells is reduced in mutant,χ2test. Three fish per genotype (three technical replicates each).eSchematic of the role of Myogenin during differentiation, fusion and growth of muscle fibres. During myogenesis, committed MPCs leave the cell cycle, begin to elongate and express early muscle-specific genes during terminal differentiation into myocytes. At this stage, Myogenin (MYOG) promotes the expression ofmyomaker(MYMK),myomixer(MYMX) andjam3b(JAM3B). These fusogenic proteins prompt myocyte fusion to form muscle fibres. In the absence of Myogenin, myocytes undergo terminal differentiation but fail to express Myog-module genes, remain mononucleated and grow less throughout life. Residual myocyte fusion inMyogmutants in the medial region of the somite (bracket) is sustained by Hedgehog (Hh) signalling Statistical analyses used GraphPad (Prism 6) for unpaired two-tailed Student’s t test or Statplus:mac v5 for ANOVA with Bonferroni or Tukey post-hoc tests to assess significant differences between mutant and sibling groups, unless otherwise stated. χ 2 test was used to analyse difference between distributions using raw values. All data are expressed as mean ± standard error of the mean (SEM). Unless otherwise stated, numbers on columns represent number of fish analysed. p values for rejection of the null hypothesis of no difference between groups are indicated above columns.